USP8 maintains embryonic stem cell stemness via deubiquitination of EPG5 Embryonic stem cells (ESCs) can propagate in an undifferentiated state indefinitely in culture and retain the potential to differentiate into any somatic lineage as well as germ cells. The catabolic process autophagy has been reported to be involved in ESC identity regulation, but the underlying mechanism is still largely unknown. Here we show that EPG5, a eukaryotic-specific autophagy regulator which mediates autophagosome/lysosome fusion, is highly expressed in ESCs and contributes to ESC identity maintenance. We identify that the deubiquitinating enzyme USP8 binds to the Coiled-coil domain of EPG5. Mechanistically, USP8 directly removes non-classical K63-linked ubiquitin chains from EPG5 at Lysine 252, leading to enhanced interaction between EPG5 and LC3. We propose that deubiquitination of EPG5 by USP8 guards the autophagic flux in ESCs to maintain their stemness. This work uncovers a novel crosstalk pathway between ubiquitination and autophagy through USP8-EPG5 interaction to regulate the stemness of ESCs. Autophagy is a highly conserved lysosome-mediated catabolic process in eukaryotic cells [1] , [2] , [3] . It was first defined as a bulk degradation process that generates resources to meet the cell’s requirements for metabolites and energy under stress conditions [4] , [5] . However, increasing numbers of studies have indicated that basal autophagy acts as a critical process to maintain cellular homeostasis by removing misfolded or aggregation-prone proteins and damaged organelles [6] , [7] , [8] . Recently, significant progress was achieved in understanding the function of autophagy in stem cell regulation. In adult stem cells, increasing evidence suggests that autophagy is not only critical for enhancing the ability to resist stress conditions but is also essential for self-renewal and differentiation [9] , [10] , [11] , [12] , [13] . Adult stem cells, for example hematopoietic stem cells (HSCs), rely on basal autophagy to clear the active and healthy mitochondria, thereby keeping their metabolic rate low in order to maintain a quiescent pool [9] . In contrast, embryonic stem cells (ESCs) maintain a high autophagic flux to ensure a fast metabolic rate for rapid proliferation and self-renewal [14] . In addition, basal autophagy has been identified to degrade the mitochondria in mouse ESCs, thus maintaining mitochondrial homeostasis. In Atg3 -knockout ESCs, dysfunctional autophagy inhibits mitochondrial removal, resulting in accumulation of the abnormal mitochondria and attenuated pluripotency [15] . These data suggest that high autophagic flux is an ESC-intrinsic characteristic and plays critical roles in ESC self-renewal and pluripotency. Thus, the molecules that promote autophagy may be beneficial for the maintenance of ESC pluripotency. To this end, we perform a screen for molecules that promote autophagy in mouse ESCs and identify EPG5, a metazoan-specific autophagy regulator, as a new guardian of ESC stemness. Moreover, using the coiled-coil domain of EPG5 as a bait, we define a novel EPG5-interacting protein, USP8, which is highly expressed in ESCs and guards ESC identity through deubiquitination of EPG5. EPG5 is essential for ESC self-renewal and pluripotency We first screened the expression of a panel of autophagy-regulatory genes in somatic cells and ESCs using existing transcriptome data as previously described, and found that EPG5 is highly expressed in ESCs [14] , [16] . EPG5, a metazoan-specific autophagy protein, regulates autophagy by promoting fusion of autophagosomes with lysosomes and/or late endosomes [17] , [18] , [19] . Using quantitative PCR and western blot assays, we confirmed that Epg5 is highly expressed in mouse ESCs at both the mRNA and protein levels compared with mouse embryonic fibroblasts (MEFs) (Fig. 1a, b ). In addition, we detected that Epg5 is highly expressed in iPSC in comparation with mouse tail fibroblast (TIF) and neuron stem cells (NSC) (Supplementary Figure 6c ). The expression of Epg5 is gradually decreased upon embryoid body differentiation (Supplementary Figure 6d ). 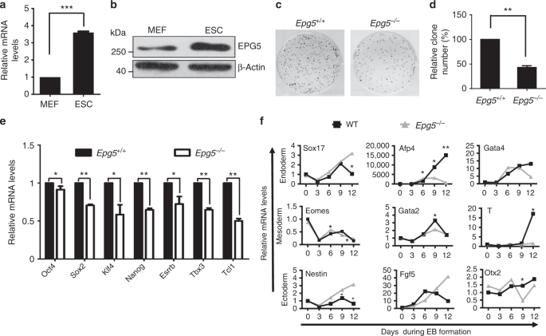Fig. 1 EPG5 maintains ESC self-renewal and pluripotency.aThe mRNA expression ofEpg5in ESCs and MEFs. Error bars indicate the standard deviation (SD) (n= 3). Three independent biological replicates. ***P< 0.001 by unpaired two-tailed Student’sttest.bWestern blot analysis of whole-cell extracts from MEFs and ESCs. β-Actin served as a loading control. Images are representative of three independent experiments.c,dColony-formation assay ofEpg5+/+andEpg5−/−ESCs. Colonies formed by ESCs were stained with alkaline phosphatase (AP). Error bars indicate the SD (n= 5). Five independent biological replicates. **P< 0.01 by unpaired two-tailed Student’sttest.eESC pluripotency is impaired byEpg5depletion. The relative mRNA expression of pluripotency genes inEpg5+/+andEpg5−/−ESCs was detected by quantitative PCR. Error bars indicate the SD (n= 3). Three independent biological replicates. **P< 0.01, *P< 0.05 by unpaired two-tailed Student’sttest.fAbsence of EPG5 impairs ESC lineage specification. The relative mRNA expression levels of genes representative of the ectoderm, mesoderm, and endoderm were detected during embryonic body (EB) differentiation by quantitative PCR on the indicated days. Data shown are representative of three independent experiments. Error bars indicate the SD (n= 4). Four independent biological replicates. **P< 0.01, *P< 0.05 by two-way ANOVA with Bonferroni’s correction (WT compared withEpg5−/−) The Epg5 expression in human pluripotent stem cells like ESC and iPSC is higher than that of human somatic cells as well (Supplementary Figure 10a ). To investigate whether EPG5 is involved in the regulation of ESC identity, we designed specific small interfering RNAs (siRNAs) targeting Epg5 and found that transient inhibition of Epg5 leads to ESC differentiation and reduced expression of pluripotency genes in both mouse and human ESCs (Supplementary Figure 1 a– d , Supplementary Figure 10 b, 10c ). 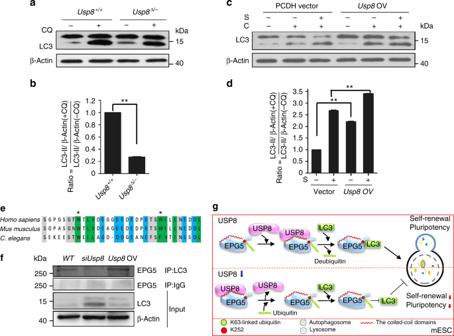Fig. 6 USP8 dynamically regulates the EPG5-LC3 interaction.aWestern blotting for LC3 and β-actin inUsp8+/+andUsp8▵/−ESCs. β-Actin served as the loading control. Cells were treated with 50 μM chloroquine (CQ) for 2 h.bQuantification of autophagic flux inaby calculating the ratio of LC3-II with or without CQ treatment. Error bars indicate the SD (n= 3). Three independent biological replicates. **P< 0.01 by unpaired two-tailed Student’sttest.cWestern blotting for LC3 and β-actin in WT andUsp8-overexpression stable ESCs upon nutrient deprivation. β-Actin served as the loading control. Cells were treated with 50 μM chloroquine (C) for 2 h and/or starved (S) in EBSS for 2 h.dQuantification of autophagic flux by calculating the ratio of LC3-II with or without CQ treatment inc. Error bars indicate the SD (n= 3). Three independent biological replicates. **P< 0.01 by unpaired two-tailed Student’sttest.eSequence alignment of the LC3-binding region (LIR) in human, mouse, and C. elegans EPG5 proteins. The aromatic residues in the two LIR motifs are indicated by asterisks. Conserved hydrophilic residues are in gray, conserved hydrophobic residues are in green, and conserved negatively charged residues are in blue.fLysates ofUsp8-overexpression and siUsp8-knockdownESCs were immunoprecipitated with anti-LC3 or anti-IgG and immunoblotted with anti-EPG5 and anti-IgG antibodies. Input cell lysates were immunoblotted with anti-LC3 and anti-actin antibodies as controls. Cells were starved for 2 h before analysis.gA proposed model of the role of the USP8-EPG5-LC3 pathway in regulating ESC stemness Fig. 1 EPG5 maintains ESC self-renewal and pluripotency. a The mRNA expression of Epg5 in ESCs and MEFs. Error bars indicate the standard deviation (SD) ( n = 3). Three independent biological replicates. *** P < 0.001 by unpaired two-tailed Student’s t test. b Western blot analysis of whole-cell extracts from MEFs and ESCs. β-Actin served as a loading control. Images are representative of three independent experiments. c , d Colony-formation assay of Epg5 +/+ and Epg5 − / − ESCs. Colonies formed by ESCs were stained with alkaline phosphatase (AP). Error bars indicate the SD ( n = 5). Five independent biological replicates. ** P < 0.01 by unpaired two-tailed Student’s t test. e ESC pluripotency is impaired by Epg5 depletion. The relative mRNA expression of pluripotency genes in Epg5 +/+ and Epg5 − / − ESCs was detected by quantitative PCR. Error bars indicate the SD ( n = 3). Three independent biological replicates. ** P < 0.01, * P < 0.05 by unpaired two-tailed Student’s t test. f Absence of EPG5 impairs ESC lineage specification. The relative mRNA expression levels of genes representative of the ectoderm, mesoderm, and endoderm were detected during embryonic body (EB) differentiation by quantitative PCR on the indicated days. Data shown are representative of three independent experiments. Error bars indicate the SD ( n = 4). Four independent biological replicates. ** P < 0.01, * P < 0.05 by two-way ANOVA with Bonferroni’s correction (WT compared with Epg5 − / − ) Full size image We then designed an sgRNA targeting the first exon of the mouse Epg5 gene and knocked out Epg5 in ESCs using the CRISPR-Cas9 system (Supplementary Figure 1e ). Western blotting confirmed the absence of EPG5 protein expression in Epg5 -knockout ( Epg5 −/− ) ESCs (Supplementary Figure 1f ). Furthermore, the Epg5 −/− ESCs have a normal karyotype (Supplementary Figure 1g ). Using colony-formation assays, we found that depletion of Epg5 in ESCs significantly inhibited the colony-formation efficiency compared with wild-type (WT) ESCs (Fig. 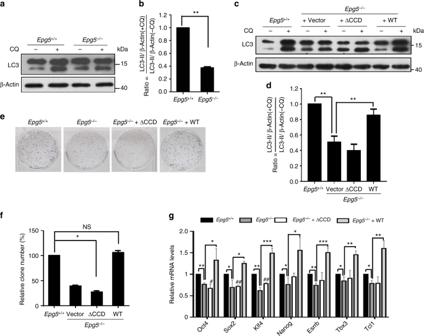1c, d ). Fig. 2 EPG5 depends on its coiled-coil domain to regulate ESC identity.aWestern blotting for LC3 and β-actin inEpg5+/+andEpg5−/−ESCs. β-Actin served as a loading control. Samples were treated with or without the autophagy inhibitor chloroquine (50 μM) for 2 h. Images are representative of three independent experiments.bQuantification of autophagic flux inaby calculating the ratio of LC3-II with or without CQ treatment. Error bars indicate the SD (n= 3). Three independent biological replicates. **P< 0.01 by unpaired two-tailed Student’sttest.cIntroduction of wild-typeEpg5but not anEpg5mutant lacking the coiled-coil domain (∆CCD) intoEpg5−/−cells ameliorates the impaired autophagic flux.dQuantification of the autophagic flux by calculating the ratio of LC3-II with or without CQ treatment inc. Error bars indicate the SD (n= 3). Three independent biological replicates. **P< 0.01 by unpaired two-tailed Student’sttest.e,fIntroduction of WTEpg5but not the ∆CCDEpg5mutant intoEpg5−/−cells restored the colony-formation ability. ESC colonies were stained with AP. Error bars indicate the SD (n= 3). Three independent biological replicates. NS not significant. *P< 0.05 by unpaired two-tailed Student’sttest.gReduced pluripotency gene expression inEpg5−/−ESCs is rescued by introduction of WTEpg5but not the ∆CCDEpg5mutant. Error bars indicate the SD (n= 3). Three independent biological replicates. *P< 0.05, **P< 0.01, ***P< 0.001,#P< 0.05,##P < 0.01 by unpaired two-tailed Student’s t test. # (Epg5-/-+∆CCD compared with Epg5+/+) Epg5 deletion did not affect ESC apoptosis and expression of differentiation marker genes (Supplementary Figure 2 a, b and Supplementary Figure 9 ). These results indicated that EPG5 is essential for ESC self-renewal. To test whether loss of EPG5 affects ESC pluripotency, we assessed the mRNA expression of pluripotency genes by quantitative PCR. We found that pluripotency gene expression was reduced in Epg5 −/− versus Epg5 +/+ ESCs, suggesting that depletion of Epg5 leads to compromised pluripotency in ESCs (Fig. 1e ). In support of this hypothesis, Epg5 −/− ESCs showed abnormal embryonic body (EB) differentiation, characterized by delayed expression of certain mesodermal marker genes (Fig. 1f ). Together, these data suggest that EPG5 is a critical regulator of ESC pluripotency. The coiled-coil domain of EPG5 regulates ESC identity To investigate how EPG5 regulates ESC pluripotency, we first determined whether EPG5 regulates autophagic flux, since high autophagic flux has been shown to maintain ESC self-renewal and pluripotency [14] . We detected the autophagic flux by measuring LC3-II turnover or degradation of EGFP-LC3 or colocalization of LC3 with LAMP1 in cells that were either treated or untreated with the autophagy inhibitor chloroquine. The results showed that depletion of EPG5 significantly decreased autophagic flux in ESCs (Fig. 2a, b ; Supplementary Figure 8 a– e ). We then performed bioinformatic analysis and found that EPG5 has a coiled-coil domain, which is a highly versatile protein-folding motif that can act as a recognition system for cellular signal transduction and provide mechanical stability to cells, as well as carrying out other important functional tasks [20] , [21] , [22] . To investigate whether the coiled-coil domain of EPG5 regulates autophagic flux and thus ESC identity, gain-of-function assays were performed by introducing either WT Epg5 or an Epg5 mutant lacking the coiled-coil domain (∆CCD) into Epg5 −/− ESCs (Supplementary Figure 6a ). We found that expressing WT Epg5 but not the ∆CCD Epg5 mutant in Epg5 −/− ESCs restored the decreased autophagic flux and ameliorated the defective self-renewal and pluripotency (Fig. 2c–g ). Taken together, these data provide evidence that the coiled-coil domain of EPG5 is critical for ESC identity maintenance. Fig. 2 EPG5 depends on its coiled-coil domain to regulate ESC identity. a Western blotting for LC3 and β-actin in Epg5 +/+ and Epg5 − / − ESCs. β-Actin served as a loading control. Samples were treated with or without the autophagy inhibitor chloroquine (50 μM) for 2 h. Images are representative of three independent experiments. b Quantification of autophagic flux in a by calculating the ratio of LC3-II with or without CQ treatment. Error bars indicate the SD ( n = 3). Three independent biological replicates. ** P < 0.01 by unpaired two-tailed Student’s t test. c Introduction of wild-type Epg5 but not an Epg5 mutant lacking the coiled-coil domain (∆CCD) into Epg5 − / − cells ameliorates the impaired autophagic flux. d Quantification of the autophagic flux by calculating the ratio of LC3-II with or without CQ treatment in c . Error bars indicate the SD ( n = 3). Three independent biological replicates. ** P < 0.01 by unpaired two-tailed Student’s t test. e , f Introduction of WT Epg5 but not the ∆CCD Epg5 mutant into Epg5 − / − cells restored the colony-formation ability. ESC colonies were stained with AP. Error bars indicate the SD ( n = 3). Three independent biological replicates. NS not significant. * P < 0.05 by unpaired two-tailed Student’s t test. g Reduced pluripotency gene expression in Epg5 − / − ESCs is rescued by introduction of WT Epg5 but not the ∆CCD Epg5 mutant. Error bars indicate the SD ( n = 3). Three independent biological replicates. * P < 0.05, ** P < 0.01, *** P < 0.001, # P < 0.05, ## P < 0.01 by unpaired two-tailed Student’s t test. # (Epg5 -/- +∆CCD compared with Epg5 +/+ ) Full size image EPG5 directly interacts with USP8 The coiled-coil domain of EPG5 is conserved in mammals (Fig. 3a ). 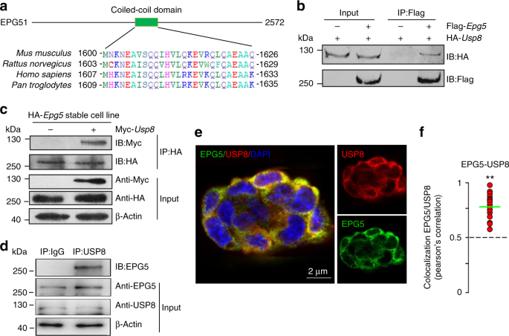To investigate the molecular mechanisms that regulate EPG5 and thus the pluripotency of ESCs, we synthesized a peptide corresponding to the coiled-coil motif of mouse EPG5 and used it as a bait to trap EPG5-interacting proteins. Fig. 3 EPG5 directly interacts with USP8 through its coiled-coil motif.aSequence alignment of the EPG5 coiled-coil domain in mouse, rat, human, and chimpanzee.bUSP8 interacts with EPG5 in HEK293T cells transfected with HA-USP8 and/or Flag-EPG5.cEPG5 interacts with USP8 in stable ESC lines harboring HA-EPG5 and/or Myc-USP8 vectors.dEndogenous EPG5 is coimmunoprecipitated with USP8 in ESCS.eConfocal fluorescence microscopy images showing that endogenous EPG5 (green) co-localizes with USP8 (red) in ESCs. DAPI (blue).fPearson’s correlation illustrated EPG5-USP8 colocalization. Red plots show colocalization values for individual cells, for >20 cells per condition. In all cases, similar results were seen in three independent experiments. Scale bars: 2 μm. **P< 0.01 by unpaired two-tailed Student’sttest inf LC-MS/MS analysis identified nine coiled-coil domain-interacting proteins with more than 13 peptide reads (Supplementary Figure 3 a, b ). One of the nine identified proteins is USP8, a deubiquitinating enzyme previously implicated in mitochondrial quality control, endosomal trafficking, and cellular proliferation [23] , [24] , [25] , [26] . To examine whether USP8 binds to EPG5 in cells, we transfected Flag-tagged Epg5 and/or HA-tagged Usp8 in HEK293T cells and performed coimmunoprecipitation (co-IP) assays. The results showed that USP8 is immunoprecipitated by EPG5, indicating that there is an interaction between EPG5 and USP8 (Fig. 3b ). To further confirm that EPG5 interacts with USP8 in ESCs, stable ESC lines harboring HA- Epg5 or Myc- Usp8 vectors were established. Co-IP assay confirmed the interaction between EPG5 and USP8 in ESCs (Fig. 3c ). Then, by using anti-USP8 antibody, we found that endogenous EPG5 can be immunoprecipitated by USP8 as well in ESCs (Fig. 3d ). Furthermore, immunofluorescence microscopy showed that EPG5 did directly interact with USP8 in ESCs (Fig. 3e, f ). These data support that EPG5 binds to USP8. Fig. 3 EPG5 directly interacts with USP8 through its coiled-coil motif. a Sequence alignment of the EPG5 coiled-coil domain in mouse, rat, human, and chimpanzee. b USP8 interacts with EPG5 in HEK293T cells transfected with HA-USP8 and/or Flag-EPG5. c EPG5 interacts with USP8 in stable ESC lines harboring HA-EPG5 and/or Myc-USP8 vectors. d Endogenous EPG5 is coimmunoprecipitated with USP8 in ESCS. e Confocal fluorescence microscopy images showing that endogenous EPG5 (green) co-localizes with USP8 (red) in ESCs. DAPI (blue). f Pearson’s correlation illustrated EPG5-USP8 colocalization. Red plots show colocalization values for individual cells, for >20 cells per condition. In all cases, similar results were seen in three independent experiments. Scale bars: 2 μm. ** P < 0.01 by unpaired two-tailed Student’s t test in f Full size image USP8 is required for regulating ESC identity We next asked whether USP8 functions in ESCs. We performed western blot assays and found that USP8 is highly expressed in both mouse and human pluripotent stem cells (including ESCs and induced pluripotent stem cells) compared with somatic cells like mouse embryonic fibroblast (MEF), TIF, neuron stem cell (NSC), and human fibroblast (HEF), foreskin (FS) cells, respectively (Fig. 4a, b ; Supplementary Figures 6 c, 10a ). We then performed RNAi assays using siRNAs targeting both mouse and human Usp8 gene. We found that decreasing the expression of Usp8 leads to ESC differentiation and lower expression of pluripotency genes (Supplementary Figures 3 c– e , 10 b, 10d ). To further investigate how USP8 affects ESC identity, we aimed to generate Usp8- knockout ESC lines by CRISPR-Cas9-mediated gene targeting (Supplementary Figure 3f ). Interestingly, we did not obtain Usp8 double-knockout ES lines within the 60 positive lines harboring indels, indicating that loss of total Usp8 may be lethal (Supplementary Figure 3g ). Then we used an ES line, which has a 12 base deletion in one allele and a 13 base deletion in another allele ( Usp8 ▵ / − ), for further analysis. These Usp8 ▵ / − ESCs have a decreased USP8 protein expression and a normal karyotype (Supplementary Figures 3 h and 6b ). Colony-formation assays were then employed to investigate the effects of USP8 on ESC self-renewal. In contrast to the WT ESCs, Usp8 ▵ / − ESCs formed a significantly lower number of colonies (Fig. 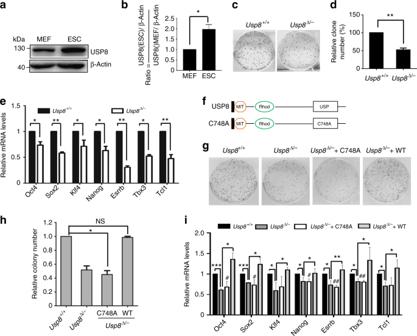4c, d ). Fig. 4 The deubiquitin activity of USP8 is required for ESC identity maintenance.a,bWestern blot analysis of whole-cell extracts from MEFs and ESCs using anti-USP8 antibody. β-Actin served as a loading control. Images are representative of three independent experiments. Error bars indicate the SD (n= 3). Three independent biological replicates. *P< 0.05 by unpaired two-tailed Student’sttest.c,dColony-formation assay ofUsp8+/+andUsp8▵/−ESCs. ESC colonies were stained by AP. Error bars indicate the SD (n= 3). Three independent biological replicates. **P< 0.01 by unpaired two-tailed Student’sttest.eESC pluripotency is impaired by decrease ofUsp8. The relative mRNA expression of pluripotency genes inUsp8+/+andUsp8▵/−ESCs was assayed by quantitative PCR. Error bars indicate the SD (n= 3). Three independent biological replicates. *P< 0.05; **P< 0.01 by unpaired two-tailed Student’sttest.fSchematic illustration of the domain organization of USP8 and the location of the C748A mutation. Boundaries of individual domains and the amino acid numbering of the catalytic Cys residue are indicated according to mouse USP8. USP, ubiquitin-specific protease domain with catalytic Cys 748. MIT-Rhod (amino acid residues 1–319).g,hThe reduced colony formation ability ofUsp8▵/−ESCs is rescued by introduction of WTUsp8, but not the C748AUsp8mutant. Error bars indicate the SD (n= 3). Three independent biological replicates. NS not significant. *P< 0.05 by unpaired two-tailed Student’sttest.iIntroduction of WT but not the C748AUsp8mutant intoUsp8▵/−cells restores the expression of pluripotency genes. The relative mRNA expression of pluripotency genes was determined by quantitative PCR. Error bars indicate the SD (n= 3). Three independent biological replicates. NS not significant. *P< 0.05, **P< 0.01, ***P< 0.001,#P < 0.05,##P < 0.01 by unpaired two-tailed Student’s t test. # (Usp8∆/-+∆C748A compared with Usp8+/+) Decreasing USP8 did not affect ESC apoptosis (Supplementary Figure 4 a, 4b ). These data indicate that USP8 is critical for ESC self-renewal. Furthermore, the reduced expression of pluripotent genes in Usp8 ▵ / − versus WT ESCs suggests the involvement of USP8 in pluripotency regulation in ESCs (Fig. 4e ). Taken together, these data indicated that USP8 is important for maintenance of ESC identity. Fig. 4 The deubiquitin activity of USP8 is required for ESC identity maintenance. a , b Western blot analysis of whole-cell extracts from MEFs and ESCs using anti-USP8 antibody. β-Actin served as a loading control. Images are representative of three independent experiments. Error bars indicate the SD ( n = 3). Three independent biological replicates. * P < 0.05 by unpaired two-tailed Student’s t test. c , d Colony-formation assay of Usp8 +/+ and Usp8 ▵ / − ESCs. ESC colonies were stained by AP. Error bars indicate the SD ( n = 3). Three independent biological replicates. ** P < 0.01 by unpaired two-tailed Student’s t test. e ESC pluripotency is impaired by decrease of Usp8 . The relative mRNA expression of pluripotency genes in Usp8 +/+ and Usp8 ▵ / − ESCs was assayed by quantitative PCR. Error bars indicate the SD ( n = 3). Three independent biological replicates. * P < 0.05; ** P < 0.01 by unpaired two-tailed Student’s t test. f Schematic illustration of the domain organization of USP8 and the location of the C748A mutation. Boundaries of individual domains and the amino acid numbering of the catalytic Cys residue are indicated according to mouse USP8. USP, ubiquitin-specific protease domain with catalytic Cys 748. MIT-Rhod (amino acid residues 1–319). g , h The reduced colony formation ability of Usp8 ▵ / − ESCs is rescued by introduction of WT Usp8 , but not the C748A Usp8 mutant. Error bars indicate the SD ( n = 3). Three independent biological replicates. NS not significant. * P < 0.05 by unpaired two-tailed Student’s t test. i Introduction of WT but not the C748A Usp8 mutant into Usp8 ▵ / − cells restores the expression of pluripotency genes. The relative mRNA expression of pluripotency genes was determined by quantitative PCR. Error bars indicate the SD ( n = 3). Three independent biological replicates. NS not significant. * P < 0.05, ** P < 0.01, *** P < 0.001, # P < 0.05, ## P < 0.01 by unpaired two-tailed Student’s t test. # (Usp8 ∆/- +∆C748A compared with Usp8 +/+ ) Full size image Previous studies reported that the C748A mutant of USP8 had markedly reduced deubiquitinase activity and failed to deubiquitinate the substrates of USP8 [24] . To investigate whether the aberrant self-renewal and pluripotency of Usp8 ▵ / − ESCs were directly caused by the decrease of USP8 deubiquitinating activity, gain-of-function assays were performed by introducing a Usp8 expression constructs into Usp8 ▵ / − ESCs. We established stable Usp8 ▵ / − ESC lines carrying WT Usp8 or the deubiquitinase-dead mutant of Usp8 (C748A) (Fig. 4f ). The colony-forming ability of Usp8 ▵ / − ESCs was rescued in stable Usp8 ▵ / − ESC lines carrying WT Usp8 , but not the C748A mutant Usp8 (Fig. 4g, h ). Similarly, the decreased expression of pluripotent genes in Usp8 ▵ / − ESC lines was restored by WT Usp8 , but not the C748A mutant (Fig. 4i ). Together, these data suggested that USP8 depends on its deubiquitinase activity to regulate the self-renewal and pluripotency of ESCs. USP8 deubiquitinates EPG5 by removing K63-ubiquitin chains To test whether USP8 deubiquitinates EPG5, we examined the ubiquitination levels in either Usp8 -overexpression or Usp8 ▵ / − ESCs. When we overexpressed Usp8 in ESCs, the ubiquitin modification of EPG5 decreased, while reduced Usp8 expression increased EPG5 ubiquitination (Fig. 5a, b ). These data indicate that USP8 deubiquitinates EPG5. To further confirm this hypothesis, we transfected Flag- Epg5 , HA- Ubiquitin , and Myc- Usp8 or Myc- Usp8 (C748A) into HEK293T cells and performed coimmunoprecipitation assays. 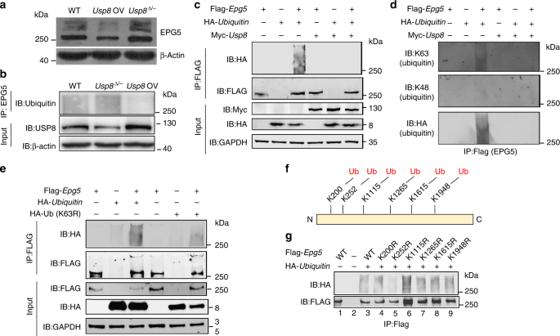The results showed that the extensive ubiquitination of EPG5 was completely abolished by overexpressing WT, but not C748A mutant Usp8 (Fig. Fig. 5 USP8 deubiquitinates the EPG5.aWestern blot analysis of whole-cell extracts from WT,Usp8-overexpression andUsp8▵/−ESC lines using anti-EPG5 antibody. β-Actin served as a loading control. Images are representative of three independent experiments.bLysates from WT,Usp8-overexpression andUsp8▵/−ESC lines were immunoprecipitated with anti-EPG5 and immunoblotted with anti-ubiquitin. Input cell lysates were immunoblotted with anti-USP8 and β-actin as controls.cLysates of HEK293T cells transfected with plasmids encoding Flag-Epg5, HA-Ubiquitinand Myc-Usp8were immunoprecipitated with anti-Flag and immunoblotted with anti-HA and anti-FLAG. Input cell lysates were immunoblotted with anti-Myc, anti-HA, and anti-GAPDH as controls.dLysates of HEK293T cells transfected with plasmids encoding Flag-Epg5, HA-Ubiquitin, and Myc-Usp8were immunoprecipitated with anti-Flag and immunoblotted with anti-K63, anti-K48, and anti-HA antibodies.eLysates of HEK293T cells transfected with plasmids encoding Flag-Epg5, HA-Ubiquitin, or HA-Ubiquitin(K63R) were immunoprecipitated with anti-Flag and immunoblotted with anti-HA and anti-FLAG antibodies. Input cell lysates were immunoblotted with anti-FLAG, anti-HA and anti-GAPDH antibodies as controls.fProteins from ESCs expressing Flag-Epg5were analyzed by LC-MS/MS mass spectrometry. Ubiquitination sites identified on EPG5 are indicated.g)Immunoblot analysis of protein extracts of HEK293T cells transfected with HA-Ubiquitintogether with plasmids expressing WT Flag-Epg5or K200R, K252R, K1115R, K1265R, K1615R, and K1948R mutants of Flag-Epg5 5c ; Supplementary Figure 5a ). These data suggested that USP8 directly deubiquitinates EPG5. Fig. 5 USP8 deubiquitinates the EPG5. a Western blot analysis of whole-cell extracts from WT, Usp8 -overexpression and Usp8 ▵ / − ESC lines using anti-EPG5 antibody. β-Actin served as a loading control. Images are representative of three independent experiments. b Lysates from WT, Usp8 -overexpression and Usp8 ▵ / − ESC lines were immunoprecipitated with anti-EPG5 and immunoblotted with anti-ubiquitin. Input cell lysates were immunoblotted with anti-USP8 and β-actin as controls. c Lysates of HEK293T cells transfected with plasmids encoding Flag- Epg5 , HA- Ubiquitin and Myc- Usp8 were immunoprecipitated with anti-Flag and immunoblotted with anti-HA and anti-FLAG. Input cell lysates were immunoblotted with anti-Myc, anti-HA, and anti-GAPDH as controls. d Lysates of HEK293T cells transfected with plasmids encoding Flag- Epg5 , HA- Ubiquitin , and Myc- Usp8 were immunoprecipitated with anti-Flag and immunoblotted with anti-K63, anti-K48, and anti-HA antibodies. e Lysates of HEK293T cells transfected with plasmids encoding Flag- Epg5 , HA- Ubiquitin , or HA- Ubiquitin (K63R) were immunoprecipitated with anti-Flag and immunoblotted with anti-HA and anti-FLAG antibodies. Input cell lysates were immunoblotted with anti-FLAG, anti-HA and anti-GAPDH antibodies as controls. f Proteins from ESCs expressing Flag- Epg5 were analyzed by LC-MS/MS mass spectrometry. Ubiquitination sites identified on EPG5 are indicated. g )Immunoblot analysis of protein extracts of HEK293T cells transfected with HA- Ubiquitin together with plasmids expressing WT Flag- Epg5 or K200R, K252R, K1115R, K1265R, K1615R, and K1948R mutants of Flag- Epg5 Full size image We next determined which kind of ubiquitin modification is removed by USP8. Ubiquitinated EPG5 was detected by an anti-K63, but not an anti-K48 ubiquitin antibody in HEK293T cells transfected with Epg5 and Ubiquitin , which indicates that EPG5 is conjugated with K63-ubiquitin chains (Fig. 5d ). Mutating K63 of ubiquitin to R63 dramatically decreased the ubiquitination of EPG5 (Fig. 5e ). Furthermore, the K63-ubiquitination of EPG5 was efficiently removed by WT, but not C748A mutant USP8 (Fig. 5d ; Supplementary Figure 5a ). These data indicate that EPG5 undergoes K63-linked ubiquitination and is specifically deubiquitinated by USP8. We then purified the EPG5 protein by immunoprecipitation using anti-FLAG antibody in HEK293T cells expressing Flag- Epg5 . LC-MS/MS analysis of the immunoprecipitated proteins identified six lysines in EPG5 that are potentially conjugated to ubiquitin (Fig. 5f ). We mutated each of the six lysines and transfected the mutant EPG5 proteins with HA- Ubiquitin . Co-IP assays showed that mutation of lysine 252, but not the lysine at other positions, eliminated EPG5 ubiquitination (Fig. 5g ). This indicates that EPG5 is conjugated to K63-ubiquitin chains via K252. USP8 regulates ESC identity through deubiquitinating EPG5 To test whether USP8 regulates ESC identity through EPG5 deubiquitination, we performed rescue assay by overexpression WT, △ LC3, or K252R mutant EPG5 in si Usp8 ESCs (Supplementary Figure 7 a, b ). Interestingly, we found only K252R mutant EPG5, but not WT or △ LC3 mutant EPG5, could compensate the defective colony formation and pluripotent gene expression lead by USP8 deterioration (Supplementary Figure 7 c– e ). These data support that USP8 regulates ESC self-renewal and pluripotency through deubiquitination of EPG5 at K252. USP8 regulates the interaction between EPG5 and LC3 To test how USP8 regulates stemness through EPG5, we explored whether USP8 regulates autophagic flux. In contrast to WT ESCs, Usp8 ▵ / − ESCs showed significantly lower autophagic flux, while Usp8 -overexpression ESCs had higher autophagic flux under both normal and starvation conditions (Fig. 6a–d ; Supplementary Figure 8 f, g ). These data indicate that USP8 guards autophagic flux in ESCs. Fig. 6 USP8 dynamically regulates the EPG5-LC3 interaction. a Western blotting for LC3 and β-actin in Usp8 +/+ and Usp8 ▵ / − ESCs. β-Actin served as the loading control. Cells were treated with 50 μM chloroquine (CQ) for 2 h. b Quantification of autophagic flux in a by calculating the ratio of LC3-II with or without CQ treatment. Error bars indicate the SD ( n = 3). Three independent biological replicates. ** P < 0.01 by unpaired two-tailed Student’s t test. c Western blotting for LC3 and β-actin in WT and Usp8 -overexpression stable ESCs upon nutrient deprivation. β-Actin served as the loading control. Cells were treated with 50 μM chloroquine (C) for 2 h and/or starved (S) in EBSS for 2 h. d Quantification of autophagic flux by calculating the ratio of LC3-II with or without CQ treatment in c . Error bars indicate the SD ( n = 3). Three independent biological replicates. ** P < 0.01 by unpaired two-tailed Student’s t test. e Sequence alignment of the LC3-binding region (LIR) in human, mouse, and C. elegans EPG5 proteins. The aromatic residues in the two LIR motifs are indicated by asterisks. Conserved hydrophilic residues are in gray, conserved hydrophobic residues are in green, and conserved negatively charged residues are in blue. f Lysates of Usp8 -overexpression and si Usp8-knockdown ESCs were immunoprecipitated with anti-LC3 or anti-IgG and immunoblotted with anti-EPG5 and anti-IgG antibodies. Input cell lysates were immunoblotted with anti-LC3 and anti-actin antibodies as controls. Cells were starved for 2 h before analysis. g A proposed model of the role of the USP8-EPG5-LC3 pathway in regulating ESC stemness Full size image EPG5 mediates autophagy by direct binding to LC3 using its LIR motif [19] , which is conserved in eukaryotes (Fig. 6e ). Since USP8 directly deubiquitinates EPG5 at K252, we next investigated whether deubiquitination of EPG5 by USP8 impairs the interactions between EPG5 and LC3 and eventually affects ESC stemness. We performed coimmunoprecipitation assays using an anti-LC3 antibody in either Usp8 -overexpression or Usp8 ▵ / − ESC lines. The results showed that overexpression of Usp8 enhanced the interaction between LC3 and EPG5. In contrast, inhibition of Usp8 abolished the interaction between LC3 and EPG5 (Fig. 6f ). These data support that USP8 guards autophagic flux for ESC identity maintenance by reinforcing the interaction between EPG5 and LC3. Previous studies demonstrated that autophagy contributes to somatic cell reprogramming [15] , [27] , [28] , [29] . These studies provided evidence to show that both canonical and noncanonical autophagy are executors of mitochondrial clearance during reprogramming, and are essential for acquisition of pluripotency. Recently, we determined that high autophagic flux is an intrinsic characteristic of mouse ESCs, and regulates the homeostasis of cellular organelles and proteins to maintain pluripotency [14] , [15] . Moreover, enhanced proteasome activity has been identified in human ESCs, and has been proposed to maintain an intact proteome for either self-renewal or generation of a specific cell lineage [30] . These findings strongly support the proposal that both autophagy and ubiquitin-mediated degradation pathways are critical catabolic processes in ESCs for regulation of cellular homeostasis and maintenance of ESC identity. Here, we defined a novel crosstalk pathway that links the two catabolic processes of autophagy and ubiquitination in ESCs to maintain ESC pluripotency. We revealed that the deubiquitinase USP8 maintains ESC identity by directly deubiquitinating EPG5 to consolidate the interaction between EPG5 and LC3 and sustain the normal autophagic flux for stemness maintenance (Fig. 6g ). At first, autophagy was believed to be a nonselective catabolic process; however, many lines of evidence revealed that autophagy mediates selective degradation of cellular protein aggregates and damaged organelles in conjunction with the ubiquitin modification system. Ubiquitination is a posttranslational modification process, in which ubiquitin is covalently linked to one or more lysine (K) of a substrate protein [31] . A recent study provides evidence that ubiquitin modification is a positive initiation signal for selective autophagy [8] . The autophagic adaptor protein p62 uses its ubiquitin-binding domain (UBA) and its LC3-interacting motif (LIR) to transfer this degradation signal to the lysosome [32] , [33] . In contrast, we show here that deubiquitination serves as a novel positive signal for maintenance of autophagic flux, and thus ESC identity. Consistent with this finding, a study has shown that the deubiquitinase USP19 stabilizes Beclin-1 by removing the K11-linked ubiquitin chains from Beclin-1, and positively regulates autophagy [34] . In addition, USP8-mediated removal of K6-linked Ub from Parkin has been shown to be required for efficient recruitment of Parkin to damaged mitochondria and subsequent mitophagy [26] . The K48-linked ubiquitination is generally considered as a canonical signal to target proteins for proteasomal degradation, while K63-linked ubiquitin modification is usually thought to be a signal for non-proteolytic pathways [31] , [33] , [35] . Here, we identified K63-linked ubiquitin in EPG5 was removed by USP8, indicating EPG5 is not degraded through the ubiquitination-mediated proteasomal signaling pathway. In consistent with this presumption, EPG5 is found to be degraded under nutrient deprivation, and lysosome inhibitor chloroquine but not proteinase inhibitor MG132 could stabilize EPG5 when protein synthesis is blocked (Supplementary Figure 5 b, c ). These data suggested EPG5 is degraded through autophagy in ESCs. In conclusion, we defined a novel mechanism, involving USP8 deubiquitination of EPG5, which underlies autophagy regulation in ESCs. We revealed that deubiquitination, like the reverse process of ubiquitination, can serve as a positive regulator of autophagy. Our findings thus extend our understanding of the crosstalk mechanisms and functions between autophagy and ubiquitin-mediated degradation. Cell culture and vector construction Human embryonic kidney 293T cells (HEK293T, ATCC, CRL-3216), human fibroblast (HEF [36] ), human foreskin (FS, ATCC, PCS-200–010™) and mouse embryonic fibroblast (MEF [15] ), TIF [15] cells, and neural stem cell (NSC [14] ) were cultured in the Dulbecco’s modified Eagle’s medium (DMEM) supplemented with 10% heat-inactivated fetal bovine serum, 2 mM glutamine, 1 mM sodium pyruvate, 100 μg/ml streptomycin, 100 U/ml penicillin, and 0.055 mM β-mercaptoethanol at 37 °C in 5% CO 2 . Both mouse ESCs [14] and iPSCs [14] were routinely maintained in the ESC medium (knockout DMEM with 15% heat-inactivated fetal bovine serum, 2 mM glutamine, 1 mM sodium pyruvate, 0.1 mM nonessential amino acids, 100 μg/ml streptomycin, 100 U/ml penicillin, 0.055 mM β-mercaptoethanol, and 1000 U/ml leukemia inhibitory factor). Both human ESCs [36] and iPSCs [36] were routinely maintained in the ESC medium (knockout DMEM, 2 mM glutamine (Invitrogen), 0.1 mM NEAA, 0.1 mM β-mercaptoethanol, 100 U/ml penicillin, 100 µg/ml streptomycin, and 20% knockout serum replacement). Mouse cDNA of Epg5 and Usp8 was cloned into the pCDH-CAG-mCherry lentivirus-vector. The HA, Flag or c-Myc tag was fused to the N terminus of Epg5 or Usp8 using standard cloning methods. All constructs generated were confirmed by DNA sequencing. All animal experiments were approved by the Ethics Committee in the Institute of Zoology, Chinese Academy of Sciences in accordance with the Guidelines for Care and Use of Laboratory Animals established by the Beijing Association for Laboratory Animal Science. Virus preparation and viral infection To prepare lentivirus for the knockdown experiments, HEK293T cells were transduced with the pSicoR vector and the lentivirus packaging vectors PSPAX2 and pMD2G using the calcium phosphate–DNA coprecipitation method. To prepare lentivirus for protein expression, HEK293T cells were transduced with pCDH-CAG-MCS-IRES-mCherry vectors and the packaging vectors PSPAX2 and pMD2G. Medium containing the virus was collected 48 h after transfection. The ES cells were infected in the collected viral supernatant in the presence of polybrene (8 µg/ml). siRNA design Mouse target sequences were as follows: Epg5 siRNA1: 5′-GGGACUGGUUAUUGAAUAA-3′, Epg5 siRNA2: 5′-GAGGCUCUUUAAUGUAUAU-3′, Usp8 siRNA1: 5′-GCGGGAUUCUCUAAAGAAA-3′, scramble: 5′-CUUACGCUGAGUACUUCGAAATT-3′. Human target sequences were as follows: hEpg5 siRNA: 5′-ATTGCAAGCCACCCAATTTATTT-3′, hUsp8 siRNA: 5′- CCACAGATTGATCGTACTAAATT-3′, hOct4 siRNA: 5′-AAGGAUGUGGUCCGAGUGUGG-3′, scramble: 5′-CUUACGCUGAGUACUUCGAAATT-3′. Epg5- knockout and Usp8 ▵ / − ESCs The sequences for the sgRNA targeting Epg5 were as follows: F: CACCGTGGACCGACAGCGTGCCGAA; R: AAACTTCGGCACGCTGTCGGTTCCAC. The sequences for the Usp8 sgRNA were as follows: F: CACCGTAACTTCGGTCTTCTTATTG; R: AAACCAATAAGAAGACCGAAGTTAC. After annealing, the oligos were ligated into the linearized vector px330. ESCs were transfected with this plasmid by electroporation. About 72 h after electroporation, single colonies were picked and sequenced. A region around the cutting site was amplified using the following primers: Epg5 -F, 5′-AACTGCCTTTGTATCTTTGG-3′ Epg5-R, 5′-ACTGTCTCCTGGAACTCGTG-3′. Usp8 -F, 5′-TATTTTTCAAGGTGTTTGTCCAGTT-3′ Usp8 -R, 5′-ATTCTAATTCCAACCAATGGTATCC-3′. PCR products were first digested with T7 enzyme and then sequenced to identify the knockout ESCs. Reagents and antibodies The following antibodies were used: mouse anti-ubiquitin (Santa Cruz(P4D1), sc-8017, 1:1000); rabbit anti-LC3 (Cell Signaling Technology (D11), #3868, 1:1000); mouse anti-LAMP1 (Cell Signaling Technology (D4O1S), #15665, 1:200); mouse anti–USP8 (Sigma-Aldrich (US872), SAB4200527, 1:1000); rabbit anti-EPG5 (Beiijng TDY Biotech CO., Ltd, TDY349F, 1:1000); mouse anti-actin (Sigma-Aldrich (AC-15), A5441, 1:5000); rabbit anti-HA tag (Abcam, ab9110, 1:1000); mouse anti-FLAG tag (Abmart, M20008, 1:1000); rabbit anti-Myc tag (Abmart, M20002, 1:1000); Alexa Fluor ® 488 donkey anti-rabbit IgG (H + L) (Invitrogen Thermo Fisher Scientific, A21206, 1:500); Alexa Fluor ® 555 donkey anti-mouse IgG (H + L) (Invitrogen Thermo Fisher Scientific, A21203,1: 200); Alexa Fluor ® 647 donkey anti-mouse IgG (H + L) (Invitrogen Thermo Fisher Scientific, A21235, 1:500). Chloroquine, Hoechst 33342, Baf-A1, and MG132 were obtained from Sigma-Aldrich. Colony-formation assay and AP staining ESCs were seeded at 1000 cells/well in a six-well plate, and cultured for about 7 days. The colonies were stained using an Alkaline Phosphatase Assay Kit (Beyotime), and the colony numbers were analyzed by Image-Pro Plus software. Quantitative real-time PCR Total RNA was extracted from MEFs, ESCs, and EBs with a total RNA isolation kit (GeneMark). The total RNA (2 µg) was reverse transcribed into cDNA using a SuperScript™ III First-Strand Synthesis System (Invitrogen). The primers used were as reported previously [15] and listed in Supplementary Table 1 . Immunoblotting Cells were lysed in lysis buffer (50 mM Tris-HCl [pH 7.4], 150 mM NaCl, 1% NP-40, 0.5% sodium deoxycholate, 0.1% SDS and protease inhibitor cocktail). Equivalent protein quantities were subjected to SDS-PAGE, and transferred to PVDF membranes (Millipore). Membranes were blocked with 5% nonfat milk for 1 h at room temperature and then probed with the indicated primary antibodies overnight at 4 °C, followed by the appropriate HRP-conjugated secondary antibodies for 1 h at room temperature. After washing with TBST three times, the blotted membranes were visualized with chemiluminescent kits (Millipore). Coimmunoprecipitation assay HEK293T cells or ESCs were transfected with constructs expressing Flag-Epg5 and HA-Usp8 or HA-Usp8 (C748A) using Lipofectamine 2000 (Invitrogen). Cells were lysed using lysis buffer (50 mM Tris-HCl [pH 7.4], 150 mM NaCl, 1% NP-40, 0.5% sodium deoxycholate, 0.1% SDS and protease inhibitor cocktail) 48 h after transfection. The lysates were immunoprecipitated with 2 μg of specific antibody and 30 -μl A/G agarose beads (Santa Cruz, SC-2003) overnight at 4 °C. The precipitates were washed three times with lysis buffer, and the immune complexes were boiled with loading buffer for 5 min before analysis by SDS-PAGE. Protein mass spectrometric analysis The coiled-coil domain of EPG5 was synthesized as follows: biotin-MNKNEAVSQQIHVLQKEVRQLQAE AAQ (from Beijing SciLight Biotechnology, LCC). One milligram of this short peptide was incubated with ES cells lysates followed by immunoprecipitation with anti-biotin beads. The precipitates were extensively washed with lysis buffer then boiled with SDS loading buffer and subjected to SDS-PAGE. Total proteins were excised from the gels, then subjected to in-gel digestion and analysis by LC-MS/MS. Data analysis Data are expressed as mean ± SEM. Unpaired t tests were used to analyze between-group differences. At least three independent experiments were performed in each case. Reporting Summary Further information on experimental design is available in the Nature Research Reporting Summary linked to this article.